Population genomics supports baculoviruses as vectors of horizontal transfer of insect transposons Horizontal transfer (HT) of DNA is an important factor shaping eukaryote evolution. Although several hundreds of eukaryote-to-eukaryote HTs of transposable elements (TEs) have been reported, the vectors underlying these transfers remain elusive. Here, we show that multiple copies of two TEs from the cabbage looper ( Trichoplusia ni ) transposed in vivo into genomes of the baculovirus Autographa californica multiple nucleopolyhedrovirus (AcMNPV) during caterpillar infection. We further demonstrate that both TEs underwent recent HT between several sympatric moth species ( T. ni , Manduca sexta , Helicoverpa spp. ) showing different degrees of susceptibility to AcMNPV. Based on two independent population genomics data sets (reaching a total coverage >330,000X), we report a frequency of one moth TE in ~8,500 AcMNPV genomes. Together, our results provide strong support for the role of viruses as vectors of TE HT between animals, and they call for a systematic evaluation of the frequency and impact of virus-mediated HT on the evolution of host genomes. Horizontal transfer (HT) of genetic material is the transmission of DNA between organisms by means other than parent-to-offspring inheritance. HT is pivotal to the biology and evolution of prokaryotes and is increasingly recognized as an important factor in the evolution of eukaryotes [1] , [2] , [3] . Contrasting with our detailed understanding of prokaryote-to-prokaryote HT [4] , the mechanisms and vectors underlying eukaryote-to-eukaryote HT are poorly known. Multiple events of gene HT have been characterized between eukaryotes, yet the majority of eukaryote-to-eukaryote HTs uncovered so far involve transposable elements (TEs) [5] , [6] . TEs are pieces of DNA capable of excising or copying themselves from a genomic locus, and also capable of integrating into another locus [7] . They are the single most abundant component of most eukaryotic genomes and have a profound impact on genome evolution [8] , [9] . Several hypotheses have been proposed to explain how TEs can be shuttled between eukaryotic organisms. For example, the findings of almost identical TEs in blood-sucking parasites and their vertebrate hosts suggest that host–parasite relationships can facilitate TE HTs [10] , [11] . In addition, viruses have been proposed as candidate vectors allowing DNA from one organism to be transferred to the germ line of another organism [5] , [12] . In vitro transposition of TED and IFP2 TEs from insect cells to virus was first reported in the 1980s (refs 13 , 14 ). Later, in vivo transposition of Tc1-like TEs was shown to occur from insect larvae to virus [15] , [16] . These early studies demonstrated that viruses can receive a genetic load from eukaryotes and highlighted the potential of viruses in mediating TE HT between host organisms. In the past few years, the identification of a few TEs embedded in viral genomes [17] , [18] or in sequences packaged in viral particles of polydnaviruses [19] , [20] , [21] , [22] , [23] has sparked a renewed interest in the old hypothesis that viruses may act as vectors of TE HT. However, in these studies, either the donor species from which the TE likely originated was identified but the TE was not found in any putative receiving organism [17] , or the potential receiving organisms were identified but no evidence was provided showing that the TE is present in the putative donor genome [22] . To date, no single example has been reported of a TE for which additive evidence exists that it is able to naturally (that is, in vivo ) transpose in a viral genome, and that it has experienced HT in the field between potential donor and receiving organisms naturally interacting with the virus in an ecologically relevant setting. In this study, we examine populations of the baculovirus Autographa californica multiple nucleopolyhedrovirus (AcMNPV), obtained by in vivo infection of cabbage looper ( T. ni ) caterpillars. We assess the capacity of this large DNA virus to facilitate TE HT and we explore the conditions that foster virus-mediated TE HT. We demonstrate that at least two DNA transposons transpose in vivo in AcMNPV at appreciable frequency (one insertion in ~8,500 viral genomes), and that both DNA transposons have recently experienced HT in nature between insect species exhibiting varying degrees of susceptibility to AcMNPV, thereby forming plausible pairs of TE donor and receiving species. In vivo transposition of two transposons in a baculovirus We reasoned that the scarcity of TEs found integrated in sequenced viral genomes does not necessarily imply that TEs rarely jump into viral genomes. Rather, we hypothesized that the frequency of viral genomes carrying a TE copy may rarely become sufficiently high in viral populations to be detected using conventional sequencing strategies that are typically based on genomic coverage <1,000X (refs 24 , 25 ). To test this hypothesis, we analysed a viral population obtained after in vivo amplification in the cabbage looper ( T. ni; see Methods) and sequenced at ultra-deep coverage. This data set (hereafter Data set 1) corresponds to 187,536X average coverage of the 134-kb genome of the baculovirus AcMNPV. 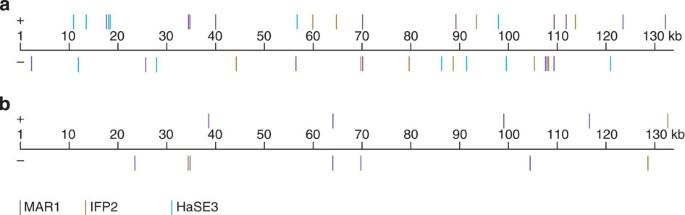Figure 1: Map of transposable element copies integrated in the genome of the AcMNPV baculovirus. Integrations took place both in the positive (+) and the negative (−) strand of the viral genome after passage of AcMNPV inT. nilarvae. (a) MAR1, IFP2 and HaSE3 insertions recovered in AcMNPV genomes sequenced at 187,536X coverage (Data set 1). (b) MAR1 and IFP2 insertions recovered in AcMNPV genomes sequenced at 145,386X total coverage (Data set 3). A first mapping of the sequencing reads onto the consensus sequences of all eukaryotic TEs available in Repbase [26] ( n =28,715 as of March 2013) yielded three TEs (MAR1, IFP2 and HaSE3) each mapped over its entire length by >180 reads ( Supplementary Table 1 ). Twenty-five additional TEs were detected, but as they were only partially mapped and supported by <10 reads, they were not considered further. To confirm that MAR1, IFP2 and HaSE3 are integrated in AcMNPV and to determine the genomic position of the various insertions, we carried out a second mapping of all reads onto these three TEs, thus allowing partially mapped reads (that is, chimeric reads containing TE and non-TE sequence) to be recovered. Inspection of the non-TE portion of the chimeric reads revealed 17, 10 and 12 distinct copies of MAR1, IFP2 and HaSE3, respectively, all integrated at different positions of the AcMNPV consensus genome sequence ( Fig. 1 , Table 1 ). Figure 1: Map of transposable element copies integrated in the genome of the AcMNPV baculovirus. Integrations took place both in the positive (+) and the negative (−) strand of the viral genome after passage of AcMNPV in T. ni larvae. ( a ) MAR1, IFP2 and HaSE3 insertions recovered in AcMNPV genomes sequenced at 187,536X coverage (Data set 1). ( b ) MAR1 and IFP2 insertions recovered in AcMNPV genomes sequenced at 145,386X total coverage (Data set 3). Full size image Table 1 Position of MAR1, IFP2 and HaSE3 insertions in the AcMNPV genome. Full size table MAR1 and IFP2 are DNA transposons that transpose via a cut-and-paste mechanism typically generating specific target site duplications (TSDs) upon insertion. Consistently, all junctions between the AcMNPV genome and the MAR1 or IFP2 elements identified in our chimeric reads corresponded to the expected TSD of the Tc1-Mariner (TA) and piggyBac (TTAA) TE superfamilies, respectively ( Supplementary Data 1 and 2 ). In addition, all TE/virus junctions identified within the chimeric reads started at the first or last nucleotide position of the MAR1 or IFP2 consensus sequences. Importantly, we selected chimeric reads encompassing five MAR1 and three IFP2 copies, and independently confirmed their integration in AcMNPV by PCR/sequencing (using the same viral genomic DNA used for ultra-deep sequencing), demonstrating that the chimeric reads that we identified are authentic TE insertions in AcMNPV, rather than sequencing artefacts (see Methods). By contrast, HaSE3, which is a short interspersed element that retrotransposes via a copy-and-paste mechanism [27] , does not generate conserved TSDs upon insertion ( Supplementary Data 3 ). Therefore, genuine retrotransposition of HaSE3 into AcMNPV could not be confidently assessed. Consequently, HaSE3 was not considered for further analysis. Altogether, our analyses of the sequence organization of chimeric reads and experimental tests demonstrate that multiple copies of at least two eukaryotic TE families became integrated in AcMNPV via bona fide transposition. The IFP2 copies we identified here correspond to the element initially characterized as an in vitro insertion in the AcMNPV genome after virus passage in a T. ni cell line [14] . IFP2 was later shown to be integrated in the genomes of T. ni and other noctuid moths [28] as well as tephritid flies [29] . It has also been widely used as a genetic tool for transgenesis and insertional mutagenesis in a broad range of organisms [30] . MAR1 has previously been described in the silkworm Bombyx mori (as MAR1_BM) and the large blue Maculinea arion (as Macmar1) [31] , [32] . We experimentally confirmed the presence of MAR1 copies in the genome of T. ni by inverse PCR and by sequencing several copies from uninfected insects (see Methods). Given the presence of the same transposons in both host and virus genomes, we formulated two hypotheses. First, the 27 IFP2 and MAR1 transposon insertions we identified in Data set 1 could result from de novo transposition of T. ni TE copies that occurred during in vivo AcMNPV infection of T. ni caterpillars. Alternatively, the transposon insertions could have been ancestrally present in the AcMNPV viral population before in vivo infection. To assess which of these two hypotheses was most likely, we analysed a second AcMNPV population data set (hereafter Data set 2) sequenced at ultra-deep coverage (163,610X), in which the viral line sequenced in the previous experiment was used for in vivo infections of beet armyworm ( Spodoptera exigua ) caterpillars. We predicted that no T. ni -like MAR1 or IFP2 insertion should be identified in viral populations amplified in S. exigua if transposons in AcMNPV result from in vivo transposition of host TE copies during viral passage (hypothesis 1), and, conversely, that if the MAR1 and IFP2 copies we found inserted into AcMNPV derive from ancestral alleles, we should be able to identify some of these copies in the AcMNPV population amplified in S. exigua (hypothesis 2). Our search did not yield any T. ni -like MAR1 or IFP2 in the S. exigua -amplified viral populations nor any other known TE. Low transpositional activity in S. exigua could explain the fact that no TE was recovered. Alternatively, our search may have missed TE insertions, as there is no TE library specifically derived from S. exigua in Repbase (or elsewhere). Anyhow, this experiment provides strong evidence that the IFP2 and MAR1 copies we identified in AcMNPV are de novo integrations resulting from in vivo transposition of T. ni TE copies that occurred during baculovirus infection. Although several TEs have previously been reported in AcMNPV under in vitro conditions [13] , [14] , [33] and in a granulovirus infecting codling moth ( Cydia pomonella ) larvae [15] , [16] , our study is the first to show that transposition does occur in vivo in AcMNPV. Recent HT of MAR1 and IFP2 To assess whether AcMNPV may have served as a vector of HT of MAR1 and IFP2 between insect species, we sought to determine the taxonomic distribution of these TEs and reconstruct their evolutionary history. In addition to B. mori and M. arion [31] , [32] , we found MAR1 in 4/8 lepidopteran species screened by PCR/sequencing ( Lomaspilis marginata , Agrotis ipsilon , S. exigua and Epicallia villica ) and in one moth species for which whole-genome sequence data are available in GenBank ( M. sexta ). Phylogenetic analyses of the MAR1 sequences yielded a tree in which the MAR1 element from AcMNPV falls within a strongly supported cluster also comprising the MAR1 copies from T. ni and M. sexta ( Fig. 2a ). 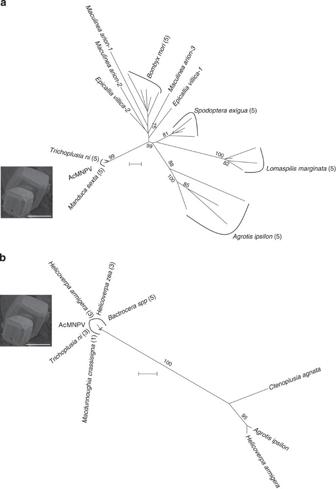Figure 2: Phylogenies of the two transposons found integrated in the AcMNPV genome. (a) Tree of MAR1 copies. Scale bar for the branch length is 0.01 substitution per site. (b) Tree of IFP2 copies. Scale bar for the branch length is 0.1 substitution per site. Bootstrap values >70% are shown on branches. The numbers of copies used for phylogenetic analysis are shown in brackets for each species. For each tree, the AcMNPV transposable element corresponds to the consensus sequence of all copies found integrated in the viral genome. The AcMNPV pictures were taken using scanning electron miscroscopy. White scale bar, 1 μm. The relationships within the cluster are unresolved because all branches are very short, reflecting the extremely low genetic distances (0.1–0.5%) separating the MAR1 copies found in these three genomes ( Table 2 ). Strikingly, the T. ni and M. sexta MAR1 copies are virtually identical despite >100 million years separating the two species [34] . Furthermore, within the T. ni and M. sexta genomes, all MAR1 copies are virtually identical (0.1–0.2% nucleotide divergence; Table 2 ). Overall, these results demonstrate that the MAR1 element we found integrated in AcMNPV has very recently been horizontally transferred between the T. ni and M. sexta lineages. Figure 2: Phylogenies of the two transposons found integrated in the AcMNPV genome. ( a ) Tree of MAR1 copies. Scale bar for the branch length is 0.01 substitution per site. ( b ) Tree of IFP2 copies. Scale bar for the branch length is 0.1 substitution per site. Bootstrap values >70% are shown on branches. The numbers of copies used for phylogenetic analysis are shown in brackets for each species. For each tree, the AcMNPV transposable element corresponds to the consensus sequence of all copies found integrated in the viral genome. The AcMNPV pictures were taken using scanning electron miscroscopy. White scale bar, 1 μm. Full size image Table 2 MAR1 inter and intra-specific distances between the various lepidopteran species in which we found these elements. Full size table Using a similar approach, we did not detect IFP2 in any species other than those in which it had previously been found [28] , [29] . Phylogenetic analyses of the IFP2 sequences yielded a tree in which the IFP2 element from AcMNPV falls within a strongly supported cluster also comprising IFP2 copies from the moths T. ni, Helicoverpa armigera , H. zea , Macdunnoughia crassisigna and the tephritid fly Bactrocera spp ( Fig. 2b ). Again, the relationships within the cluster are unresolved because of the very low genetic distances (1–5%) between the IFP2 copies found in the various genomes ( Table 3 ). Remarkably, the genetic distance between the neutrally evolving T. ni and H. zea/H. armigera IFP2 sequences (5%) is much lower than the 10.9% average distance we calculated for the 12 most conserved orthologous nuclear genes between these species (see Methods). In addition, IFP2 was not detected in Heliothis virescens [28] , which is closely related to H. zea and H. armigera , indicating that IFP2 distribution is discontinuous within noctuid moths. Furthermore, IFP2 copies are highly similar within the T. ni , H. zea and H. armigera genomes (0.4–1.7% nucleotide divergence; Table 3 ). As for MAR1, these results indicate that the IFP2 element we found integrated in AcMNPV has very recently been horizontally transferred between the T. ni and H. zea / H. armigera lineages. Table 3 IFP2 inter and intra-specific distances between the various lepidopteran species in which we found these elements. Full size table Frequency of host TEs in baculovirus populations T. ni , M. sexta , H. zea and H. armigera are widespread agricultural pests of widely overlapping geographic distributions in North America. Remarkably, all these moths can be infected by AcMNPV, even if they extensively vary in susceptibility, T. ni being highly susceptible and M. sexta being highly resistant [35] , [36] . To further evaluate the role of baculoviruses in mediating IFP2 and MAR1 HTs between insect species, we estimated the frequency of transposon insertions in the sequenced AcMNPV population. Given that the number of viral genomes used to construct the sequencing library (14 × 10 9 ) is far greater than the coverage reached by sequencing in Data set 1 (187,536X), we use the latter value as a proxy for the number of sequenced AcMNPV genomes. This yields a frequency of 27 insertions in 187,536 AcMNPV genomes, that is, 1 insertion in 6,900 AcMNPV genomes. To evaluate the reproducibility and accuracy of this estimate, we analysed ten additional AcMNPV populations (hereafter Data set 3) sequenced at ultra-deep coverage (145,386X in total). Data set 3 is derived from ten independent replicates of an experiment consisting of in vivo infections of T. ni caterpillars initiated with the AcMNPV stock used for Data set 1. Our search for TEs in Data set 3 recovered the same three TEs as in Data set 1: MAR1, IFP2 and HaSE3. In particular, we identified MAR1 or IFP2 insertions in six replicates, yielding a total of nine MAR1 and three IFP2 copies across all replicates ( Table 4 ). The 12 transposon copies from Data set 3 are all integrated at different positions of the AcMNPV consensus genome sequence, and all but one are distinct from the 27 insertions identified in Data set 1 ( Table 1 ). The near absence of overlap in the sets of insertions recovered in the independent replicates and data sets provides further evidence that the TE copies we identifiedin AcMNPV are de novo integrations originating from the T. ni host, that occurred in vivo during viral infection. When combining the ten replicates of Data set 3 together, we infer a frequency of 12 insertions in 145,386 AcMNPV genomes, that is, 1 insertion in ~12,100 AcMNPV genomes ( Table 4 ). The frequency in the six replicates in which at least one insertion was found ranges from one insertion in ~3,100 (replicate 3) to one in ~21,800 (replicate 7) viral genomes. The frequency in the four replicates in which no transposon was detected cannot be confidently assessed. However, we can conservatively infer that the frequency is lower than the observed sequencing coverage, that is, it is lower than one insertion in ~9,200, ~10,700, ~18,300 and ~8,800 viral genomes for replicates 2, 5, 8 and 9, respectively ( Table 4 ). Therefore, the frequencies in these four replicates are compatible with the range of frequencies derived from the six other replicates, as is the frequency calculated from Data set 1 (one insertion in ~6,900 viral genomes). In summary, all data sets consistently indicate a frequency of one insertion in 3,000–22,000 viral genomes, with a global estimate of one in ~8,500 when all data sets are combined ( Table 4 ). Table 4 Frequencies of MAR1 and IFP2 insertions in AcMNPV population genomics data sets. Full size table It is noteworthy that our estimate of TE frequency in AcMNPV genomes is solely based on the two transposons for which there is undisputable evidence of integration into viral genomes by bona fide transposition (IFP2 and MAR1). Should we assume bona fide retrotransposition of HaSE3 into AcMNPV, TE frequency in AcMNPV populations would substantially be increased (for example, by almost 50% based on Data set 1). Furthermore, we may have overlooked a number of TEs because we are working with moth species for which neither the genomes nor the TE libraries are readily available. We conclude that our estimate of one insertion in ~8,500 AcMNPV genomes is probably a very conservative underestimate of the true frequency. In this study, we identified two eukaryotic TEs that underwent very recent HT between several sympatric animal species. We also showed that these TEs integrated via in vivo transposition in the genome of a virus infecting these animal species at a frequency of one copy in ~8,500 genomes. Below we discuss the biological relevance of this frequency as well as other factors influencing the rate of TE HT. Interestingly, we found that transposons are over-represented in non-coding relative to coding regions of the AcMNPV genome (Khi2 test; P <0.00001; Table 1 ). This suggests that purifying selection efficiently acts on baculovirus genomes during the course of a single infection cycle, and that individual TE copies are unlikely to reach high frequency in baculovirus populations (unless they provide substantial fitness gain to the genome). Nevertheless, the AcMNPV dose that produces 50% mortality of an orally infected population of caterpillars varies from <10 to several tens of thousands of occlusion bodies (OBs) depending on the host species [37] . OBs are proteinaceous complexes allowing baculoviruses to remain viable in the environment for several years. Regarding AcMNPV, ~100 virions, each containing multiple viral genomes, are packaged in a single OB [38] . Therefore, a caterpillar typically ingests thousands to hundreds of thousands of AcMNPV genomes during infection in the wild. Therefore, even with a moderate frequency of one TE insertion in ~8,500 AcMNPV genomes, many AcMNPV infections are initiated with viral populations containing TE insertions acquired from the previous host. This implies that the opportunity for TE HT virtually exists at each baculovirus infection. Importantly, the rate of TE HT success does not only depend on the rate of TE HT opportunity. Although a single viral genome carrying a TE insertion is theoretically sufficient to enable TE HT, many factors add complexity to this picture in practice. For example, following viral infection of a new host, the TE has to be able to transpose into the host genome. This requires the TE to be competent for transposition, that is, coding and non-defective. Host-defence mechanisms may also impact the likelihood of transposition. Should transposition occur, it has to take place in the host germ line for the horizontally transferred TE to possibly experience vertical inheritance. In this context, it is interesting that, after primary infection of host midgut cells by OB-derived viruses, baculoviruses are able to mount a systemic infection in their hosts [37] , as budded viruses target virtually all tissues including gonads [39] . This opens a window of opportunity for a baculovirus-derived TE to invade the host germ line. Should transposition occur in the germ line, the viral infection has to be non-lethal to the host larvae for the invading TE to have any evolutionary fate in the new host species. With respect to AcMNPV, some species (for example, M. sexta and H. zea ) are known to be resistant, requiring high viral dose to cause death [37] . In addition, several surveys reported high levels of non-lethal baculovirus infections in adult moths [40] , [41] . This provides a favourable ground for AcMNPV-mediated TE HT to be occasionally successful. In any case, even if any single baculovirus-mediated TE HT has a remote probability to be successful, it should be kept in mind that we provide here strong evidence that a large fraction of baculovirus infections represent TE HT opportunities. Therefore, when considering the evolutionary time scale, it is very likely that many baculovirus-mediated TE HT events have been successful in nature. In conclusion, our results strongly support the role of viruses as efficient vectors of TE HT between animals. They call for a more systematic evaluation of the frequency of virus-mediated HT of DNA between animals and of its impact on host-genome evolution. Of note, the insects in which we identified recent TE HTs are agricultural pests that have undergone recent demographic expansion with the intensification of agricultural practices. Baculovirus zoonoses occur naturally in the field and are increasingly exploited for the biological control of these pests [42] . Given the frequency at which baculoviruses potentially shuttle genetic material between host species, it would be relevant to assess the impact of intensive agriculture on the recent evolution of insects. Finally, this work highlights the need to integrate the complete landscape of multitrophic interactions in which a species can be engaged to understand how its genome has evolved. Characteristics of the viral population genomics data sets We analysed three AcMNPV population genomics data sets (Data sets 1–3). The same AcMNPV stock was used to generate all three data sets. This virus was originally isolated from a single alfalfa looper ( Autographa californica ) individual collected in the field. Additional information is available elsewhere [43] . To generate Data set 1 (Genbank accession number SRS533250 ), we amplified AcMNPV through one infection cycle on cabbage looper ( T. ni ) caterpillars. Viral DNA was extracted from a solution of 1.5 × 10 10 OBs, purified by a percoll gradient pH 7.5, sucrose 0.25 M (9V of percoll/sucrose solution were added to 1V of virus solution). OBs were dissolved using Na 2 CO 3 to release nucleocapsids [44] . The bulk of contaminating bacterial and host DNA was removed by DNase digestion. Viral DNA was then extracted using the QIAamp DNA Mini kit (Qiagen). Before sequencing, contamination of viral DNA by host DNA was checked by PCR on the nuclear gene marker actin and mitochondrial gene cytochrome oxidase subunit I (COI) ( Supplementary Table 2 ). PCRs were conducted on 1 ng genomic DNA using the Goldstar PCR Mix (Eurogentec) and the following temperature cycling: initial denaturation at 95 °C for 4 min, followed by 30–35 cycles of denaturation at 94 °C for 60 s; annealing at 49–58 °C (depending on the primer set) for 60 s; and elongation at 72 °C for 60–90 s, ending with a 10-min elongation step at 72 °C. No insect-specific PCR product was amplified from the viral DNA, suggesting that host DNA contamination must be extremely low. A 2-μg aliquot of this extraction was used to construct a paired-end library (insert size 260 bp), which was sequenced on half a lane of an Illumina GAIIx platform, generating 171 million 151-bp paired reads. A 133,926-bp long AcMNPV consensus genome sequence was assembled from this data set using Newbler 2.8, and mapping of all reads onto this consensus genome sequence (using the local alignment mode of Bowtie2 (ref. 45 ) revealed an ultra-deep average coverage of 187,536X. Data sets 2 and 3 were generated by ultra-deep sequencing of AcMNPV populations passaged on S. exigua and T. ni caterpillars, respectively (Genbank accession numbers SRS534469 , SRS534534 , SRS534575 , SRS534677 , SRS534587 , SRS534590 , SRS534631 , SRS534673 , SRS536572 , SRS536571 and SRS534470 , SRS534499 , SRS534514 , SRS534536 , SRS534537 , SRS534543 , SRS534542 , SRS536937 , SRS534588 and SRS534589 ). Each data set was obtained by setting up ten replicates of an experiment consisting of ten successive in vivo infection cycles. Viral DNA from each replicate was extracted as described above and used to construct a paired-end library (insert size 265 bp), which was sequenced on a Illumina HiSeq2000 platform, generating at total of 272 and 215 million 101-bp paired reads for Data sets 2 and 3, respectively. Identification of TE insertions To detect TEs in each data set, we first mapped the sequencing reads onto consensus sequences of all eukaryotic TEs available in the Repbase reference database [26] as of 19 March 2013 ( n =28,715), using the end-to-end alignment mode of Bowtie2 (ref. 45 ). To assess whether the TEs detected using this approach were inserted in multiple copies in the sequenced viral population and to determine the genomic position of each insertion, we performed a second mapping of all reads onto the TEs identified in the first mapping using the local alignment mode of Bowtie2. The second mapping yielded several chimeric reads for which only a portion was mapped onto a given TE consensus sequence. For each chimeric read, we assessed the identity of the non-TE portion by BLASTN searches against the non-redundant nucleotide GenBank database and the aforementioned AcMNPV consensus genome. Next, we verified by PCR and Sanger sequencing that the chimeric reads were not experimental artefacts (for example, generated during library construction or sequencing). We designed primer pairs on the TE and non-TE portions of five MAR1 and three IFP2 chimeric reads from Data set 1 and carried out PCR using the original AcMNPV genomic DNA used for Illumina sequencing as a template. The list of primers we used is provided in Supplementary Table 2 . PCRs were conducted on 25 ng genomic DNA using AmpliTaq Gold (Applied Biosystems) and the following temperature cycling: initial denaturation at 95 °C for 10 min, followed by 40 cycles of denaturation at 94 °C for 30 s; annealing at 52–58 °C (depending on the primer set) for 30 s; and elongation at 72 °C for 30 s, ending with a 10-min elongation step at 72 °C. Purified PCR products were directly sequenced using ABI BigDye sequencing mix (1.4 μl template PCR product, 0.4 μl BigDye, 2 μl manufacturer supplied buffer, 0.3 μl primer and 6 μl H 2 O). Sequencing reactions were ethanol precipitated and run on an ABI 3730 sequencer. Assessment of host DNA contamination We investigated whether the chimeric reads could all derive from host contamination. The non-TE portion of three MAR1 and one IFP2 chimeric reads from Data set 1 were not mapped onto the aforementioned AcMNPV consensus genome sequence or any of the baculovirus genomes available in GenBank. We verified by PCR (as described above) the presence of these sequences in the original DNA extract used for Illumina sequencing, thus excluding the possibility that these chimeric reads result from a technical sequencing artefact. We postulated that these chimeric reads bridging TE and non-TE sequences resulted from traces of contaminating host genomic DNA that could not be completely digested before viral genomic DNA extraction. This hypothesis is supported by the fact that we were able to amplify by PCR the sequence corresponding to the IFP2 chimeric read in two non-infected T. ni individuals. However, we were not able to amplify the sequences corresponding to the three MAR1 chimeric reads in these two T. ni individuals. As we demonstrate in this study, MAR1 has invaded the T. ni genome very recently and is likely to be still actively transposing in this species. These three MAR1 chimeric reads therefore probably correspond to polymorphic loci for presence/absence of MAR1 insertions in T. ni . Given that the T. ni genome is larger than the AcMNPV genome by several orders of magnitude—known genome sizes vary from 0.38 to 1.4 gigabases for Noctuid species [46] —and that we found many more MAR1 and IFP2 chimeric reads mapping onto the AcMNPV genome ( n =27) than chimeric reads not mapping onto it ( n =4), we can confidently infer that the amount of host DNA co-extracted with the viral DNA is extremely low. In any case, host DNA contamination does not affect our results and conclusions because we assessed the viral origin of all 27 MAR1 and IFP2 chimeric reads with high confidence, as the non-TE portion of these reads is identical to its cognate region in the AcMNPV genome. Furthermore, we independently confirmed by PCR and Sanger sequencing that multiple chimeric reads are genuinely present in the population of baculovirus genomes. We are also highly confident that our TE-AcMNPV chimeric reads are not derived from TEs integrated into endogenized AcMNPV fragments located in the T. ni genome. This is because endogenization of viruses in general is rare and very few endogenous large DNA viruses (such as baculoviruses) have been reported so far [47] , [48] . Furthermore, endogenous viruses generally correspond to fragments of the genome of their cognate exogenous virus, and when present in a given genome they usually have a low copy number [47] . Finally, as the viral DNA sample we sequenced contains at most traces of contaminating host DNA and any endogenized AcMPNV fragment would represent a tiny fraction of the host genome, it is more parsimonious to conclude that TE-AcMNPV chimeric reads do not derive from contaminating host genome. And this is without considering that any endogenized AcMNPV fragment would have to have recently integrated in the T. ni genome (as all virus-like sequences in our chimeric reads were identical to the AcMNPV genome sequence) while having experienced multiple transposition events by several TEs. Sequence and phylogenetic analyses To assess the taxonomic distribution of IFP2 and MAR1 TEs observed in our baculovirus population, we used the consensus sequence of both TEs as queries in BLASTN searches against the non-redundant nucleotide and whole-genome sequence GenBank databases. We also experimentally searched for these TEs by PCR and Sanger sequencing in eight lepidopteran species ( A. ipsilon , A. gamma , Charanyca trigrammica , E. villica , L. marginata , Maniola jurtina , Spilosoma lubricipeda and S. exigua ) for which genomic DNA was available in our laboratory (primers are provided in Supplementary Table 2 ). PCRs were conducted on 100 ng genomic DNA using GoTaq (Promega) and the following temperature cycling: initial denaturation at 94 °C for 5 min, followed by 30 cycles of denaturation at 94 °C for 30 s; annealing at 55 °C for 30 s; and elongation at 72 °C for 1 min, ending with a 10-min elongation step at 72 °C. PCR products were cloned into pGEM-T easy vector (Promega) and five clones were sequenced for each species in which an element was detected (Genbank accession numbers: KJ144864 - KJ144888 ). We emphasize that a lack of PCR amplification for any given species does not prove the absence of the TE in that species, as diverged copies of the TE could have precluded amplification. Nevertheless, this would not affect our results and conclusions because we were aiming at detecting recent TE copies showing high similarity to those found in AcMNPV. As MAR1 is present in B. mori [31] and M. sexta (this study), two species for which whole-genome sequences are available, we assessed MAR1 copy number and evaluated nucleotide similarity between each copy found in the two genomes and their respective consensus sequences using RepeatMasker [49] . Given that the genomic DNA sample that has been sequenced contains traces of host DNA, and that the TEs inserted in AcMNPV are highly similar to those found in the T. ni genome, the origin (host or AcMNPV genome) of all non-chimeric reads mapping entirely onto MAR1 or IFP2 cannot confidently be assessed. For this reason, the consensus sequence reconstructed for the MAR1 and IFP2 elements inserted in the AcMNPV genome was based only on the chimeric reads for which the non-TE portion was of undisputable AcMNPV origin. These consensus sequences therefore are partial elements that include a portion of their 5′ and 3′ regions (MAR1=622 bp and IFP2=533 bp). Sequence alignments were performed using BioEdit [50] , and Jukes–Cantor-corrected intra as well as inter-species distances were calculated for each element in MEGA 5 (ref. 51 ). Inter-species distances were calculated between majority rule consensus sequences of each element reconstructed based on an alignment of three or more copies. Nucleotide alignments of all MAR1 and IFP2 sequences used are provided in Supplementary Data 4 and 5 . Phylogenetic analyses were carried out using PhyML 3.0 (ref. 52 ). Models of nucleotide evolution best fitting each alignment were determined using jModelTest2 (ref. 53 ). To assess whether IFP2 was transmitted vertically or horizontally between T. ni and H. zea / H. armigera , we calculated distances between several genes that are conserved at orthologous loci between T. ni and H. zea/H. armigera . To select these genes, we used 148 T. ni mRNA sequences encoding proteins with known function as queries in BLASTN searches against H. zea / H. armigera EST sequences. We then selected the 14 most conserved genes between the two genera according to the BLAST results and verified that these genes evolve under purifying selection using the codon based Z -test of selection implemented in MEGA 5. We finally retained 12 genes and calculated the Jukes–Cantor-corrected distances in MEGA 5: actin (5.4%), AMP deaminase (12.9%), cytoplasmic actin A3a (5.5%), ecdysone receptor (11.7%), elongation factor 1 alpha (6.6%), enolase (13.7%), heat-shock 70 protein (10.7%), nucleolar cysteine rich protein (16.5%), G protein alpha Q subunit (10.5%), translationally controlled tumour protein (10.2%), ultraspiracle protein (13.5%) and wingless (13.6%). These genes have been transmitted vertically between Trichoplusia and Helicoverpa genera and evolve under purifying selection. In animals, DNA transposons generally undergo a burst of transposition after invading a naive genome [54] , with each copy generated by this initial burst then evolving neutrally and accumulating mutations in an idiosyncratic way. This evolutionary process explains the unresolved star topologies that are typically obtained when reconstructing the phylogeny of multiple copies of a given DNA TE taken from an animal genome [10] , [55] . It is important to underline here that this pattern cannot be generalized to all TEs in all host species as for example, some animal retrotransposons and many plant TEs do not show evidence of pronounced transposition burst and are known to be composed of several functional variants that are able to transpose for long periods of time in a given host lineage [56] , [57] . However, in animals, given that DNA TEs are expected to evolve neutrally after insertion in the genome (unless they are domesticated [55] , [58] ), the distance calculated for a TE inherited vertically between the two moth genera should be larger than the distance obtained for conserved genes. Consistently, the distance we calculated for HaSE3 between T. ni and H. zea / H. armigera (15%) using sequences produced in the study by Wang et al . [27] is indeed larger than the average distance we calculated for the 12 most conserved genes (10.9%), suggesting vertical inheritance of HaSE3 in these noctuid moths. By contrast, the distance we calculated between T. ni and H . zea / H. armigera IFP2 (5%) is half that of the most conserved genes, suggesting IFP2 was horizontally transferred between species of the two genera. Importantly, we verified that IFP2 is evolving neutrally in the various moth genomes using the codon based Z -test of selection implemented in MEGA 5 on an alignment of six and ten IFP2 copies from Helicoverpa and T. ni , respectively. As expected according to Robertson [55] and Hartl et al . [58] , all P values for within-species comparisons were >0.05. Inverse PCR Because our study is the first to uncover MAR1 in T. ni , we characterized a copy of this element integrated in the T. ni genome by inverse PCR. We digested 2 μg of T. ni genomic DNA with BamHI (which does not cut the MAR1 consensus sequence), followed by ethanol precipitation and circularization of the digestion product by ligation using T4 DNA Ligase (NEB). PCR was then performed using primers designed on both ends of MAR1 in outward orientation (provided in Supplementary Table 2 ). A ~2.5-kb PCR product was then cloned into PGEM-T easy vector (Promega), and we Sanger sequenced a 776-bp fragment corresponding to the junction between the 3′ end of the MAR1 copy (133 bp) and the downstream flanking T. ni genomic region (643 bp). This MAR1 copy is identical or almost identical (average of 99.8% identity; range from 97.5 to 100%) over the 133 bp to all MAR1 copies found integrated in the baculovirus genome. Accession codes: The DNA sequences have been deposited in the GenBank nucleotide database under the accession codes SRP035399 (AcMNPV genomes), KJ144864 to KJ144888 (MAR1 sequences), SRS533250 (Data set 1), SRS534469 , SRS534534 , SRS534575 , SRS534677 , SRS534587 , SRS534590 , SRS534631 , SRS534673 , SRS536572 , SRS536571 and SRS534470 , SRS534499 , SRS534514 , SRS534536 , SRS534537 , SRS534543 , SRS534542 , SRS536937 , SRS534588 and SRS534589 (Data sets 2 and 3). How to cite this article: Gilbert, C. et al . Population genomics supports baculoviruses as vectors of horizontal transfer of insect transposons. Nat. Commun. 5:3348 doi: 10.1038/ncomms4348 (2014).